Receptor-interacting protein 140 attenuates endoplasmic reticulum stress in neurons and protects against cell death Inositol 1, 4, 5-trisphosphate receptor (IP 3 R)-mediated Ca 2+ release from the endoplasmic reticulum (ER) triggers many physiological responses in neurons, and when uncontrolled can cause ER stress that contributes to neurological disease. Here we show that the unfolded protein response (UPR) in neurons induces rapid translocation of nuclear receptor-interacting protein 140 (RIP140) to the cytoplasm. In the cytoplasm, RIP140 localizes to the ER by binding to the IP 3 R. The carboxyl-terminal RD4 domain of RIP140 interacts with the carboxyl-terminal gate-keeping domain of the IP 3 R. This molecular interaction disrupts the IP 3 R’s ‘head–tail’ interaction, thereby suppressing channel opening and attenuating IP 3 R-mediated Ca 2+ release. This contributes to a rapid suppression of the ER stress response and provides protection from apoptosis in both hippocampal neurons in vitro and in an animal model of ER stress. Thus, RIP140 translocation to the cytoplasm is an early response to ER stress and provides protection against neuronal death. Ca 2+ release mediated by the inositol 1, 4, 5-trisphosphate receptor (IP 3 R) is critical to cellular signal propagation [1] . However, uncontrolled Ca 2+ release from the endoplasmic reticulum (ER) triggered by IP 3 R dysfunction or ER stress elevates intracellular Ca 2+ concentration ([Ca 2+ ] i ) resulting in toxicity and cell death [2] . Thus, regulation of IP 3 R activity is vital to Ca 2+ homoeostasis and cell survival. Disruption of ER Ca 2+ homoeostasis contributes to cell death in the progression of neurological disease [3] , [4] . Depletion of ER Ca 2+ stores results in ER stress that evokes the unfolded protein response (UPR). Deregulation of the UPR elevates expression of CCAAT/enhancer-binding protein homologous protein (CHOP) resulting in ER-dependent apoptosis [5] . Conversely, blockade of ER Ca 2+ release by dantrolene and xestospongin C, inhibitors of ryanodine receptor (RyRs) and IP 3 Rs, respectively, prevents prion and amyloid-beta(Aβ)-induced neuronal death [6] , [7] . Furthermore, inhibition of IP 3 R-mediated Ca 2+ release attenuates ER stress and improves cell survival following sarcoendoplasmic reticulum calcium transport ATPase inhibition [8] . In mammals, there are three IP 3 R subtypes: IP 3 R1, 2 and 3. IP 3 R1 is the predominant subtype expressed in the cerebellum and hippocampus [9] , [10] . IP 3 R activity is regulated by proteins residing in the ER lumen or the cytosol [11] . Similar to other Ca 2+ channels, the functional IP 3 R exists as a tetramer. Its primary structure is divided into three domains: the NH 2 -terminal ligand-binding domain, the coupling domain and the carboxyl-terminal channel gate domain. ER Ca 2+ release through the IP 3 R channel is regulated by the actions of accessory modulating proteins that can interact with the large cytosolic regions of the ligand-binding domain and the channel gate domain under both normal and certain pathologic conditions [12] , [13] . The positive modulating proteins include neuronal calcium sensor 1, huntington and cytochrome c , which enhance channel opening and Ca 2+ release [14] , [15] . In contrast, the IP 3 R-binding protein released with IP 3 is a pseudo-ligand that suppresses the activity of IP 3 Rs by competing with IP 3 binding [16] . Moreover, the anti-apoptotic protein Bcl-2 inhibits IP 3 -dependent channel opening and Ca 2+ release by interacting with the channel gate domain and the coupling domain of the IP 3 R [17] . Blocking Ca 2+ transfer from the ER to mitochondria by IP 3 R-binding proteins, GIT1 and GIT2, attenuates cell death [18] . However, how IP 3 R is negatively regulated, which can be neuroprotective, following channel overactivation remains unclear. Receptor-interacting protein 140 (RIP140), a wide-spectrum transcription co-regulator, is highly expressed in multiple tissues including the brain [19] . Its primary physiological action is to negatively regulate hormonal control of gene activity by recruiting repressive chromatin remodelling machinery in the presence of hormones, thereby triggering hormone-elicited gene suppression [20] , [21] . Interestingly, the expression of RIP140 decreases with aging [22] . RIP140 knockout mice exhibit learning and memory deficits and increased stress responses [23] . Additionally, elevated RIP140 levels in the hippocampi of patients with Down syndrome [24] suggest physiological or pathological relevance of RIP140 in the brain. But the action of RIP140 in neurons remains unclear. In dissecting the molecular mechanisms underlying RIP140’s functions, we have systemically examined this protein in various cellular contexts and found that it is extensively modified by post-translational modifications in a context-dependent manner. These include various forms of phosphorylation [25] , lysine and arginine methylation [26] , lysine–vitamin B conjugation [27] , lysine acetylation and sumoylation [28] , [29] , and ubiquitination [30] . Most of these post-translational modifications modulate RIP140’s regulation of gene expression/chromatin remodelling in the nucleus, which is consistent with its principal activity as a transcriptional co-regulator. However, a novel signalling pathway rapidly stimulates the export of RIP140 from the nucleus to the cytoplasm where it then becomes a cytosolic regulator. This pathway is triggered by specific serine phosphorylation on Ser 102 and Ser 1003 followed by arginine methylation on Arg 240 , Arg 650 and Arg 948 [30] . In adipocytes, cytosolic RIP140 can interact with AS160, an Akt substrate, to suppress glucose transporter 4 and adiponectin vesicle trafficking, thereby reducing glucose uptake and adiponectin secretion [31] . Considering the high levels of neuronal RIP140 expression, the behavioural phenotypes of RIP140 knockout mice, and the gradual decline of RIP140 in aging brain, we hypothesized that RIP140 is important for the proper function of neurons. In this study, we observed rapid stress-induced export of RIP140 from the nucleus to the cytosol in neurons. The cytosolic RIP140 is an early, neuroprotective IP 3 R-interacting protein. By binding to IP 3 R to suppress its channel opening, cytosolic RIP140 helps to attenuate IP 3 R-mediated Ca 2+ release. We also demonstrate the physiological relevance of this mechanism in ER stress models in vitro and in vivo . ER stress triggers RIP140 nuclear export and ER localization RIP140 is exported from the nucleus to the cytoplasm of adipocytes following sequential post-translational modifications initiated by PKCε-dependent phosphorylation [32] . We found that in neurons, the UPR triggered the translocation of RIP140 to the cytoplasm. We applied several in vitro ER stress inducers to hippocampal neurons. Thapsigargin (Tg) depletes ER Ca 2+ by blocking ER membrane Ca 2+ pumps; dithiothreitol is a reducing agent; brefeldin A induces ER stress by collapse of the Golgi into the ER; and tunicamycin inhibits N -linked glycosylation. Treating mouse hippocampal neural cells (HT22 cells) with Tg, dithiothreitol or brefeldin A increased cytoplasmic RIP140 levels while simultaneously decreasing nuclear RIP140 levels ( Fig. 1a–c ). Aβ neurotoxicity involves elevated ER stress [33] . Interestingly, RIP140 translocation can also be triggered by aggregated Aβ peptide (Aβ 1-40 and Aβ 1-42 ) in hippocampal neurons. As shown in Fig. 1d , using lentivirus carrying green fluorescent protein (GFP)–RIP140, we detected GFP–RIP140 mainly in the nucleus, which was translocated to the cytoplasm following Aβ treatment for 24 h. To rule out the potential translational effect on the elevation of RIP140 in the cytoplasm, we applied a translational inhibitor cycloheximide. Fig. 1e,f shows that pretreatment of cells with cycloheximide did not block the increase of RIP140 in the cytoplasm. Since nuclear export of RIP140 could be triggered by PKCε-initiated phosphorylation of RIP140, we examined the effects of Tg on RIP140 (CN), a mutant previously shown defective in nuclear export in adipocytes [34] . We also employed a PKC inhibitor to examine whether this PKC pathway was involved in nuclear export of RIP140 in the stressed neurons. 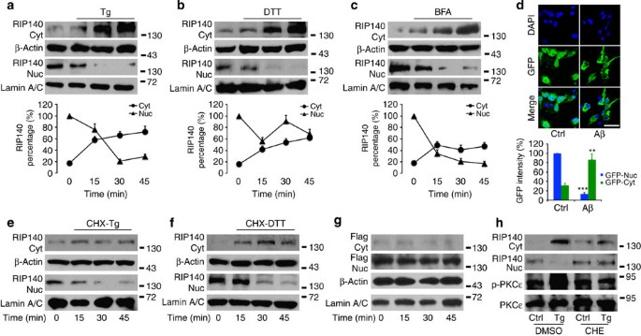Figure 1: UPR induces RIP140 translocation to cytoplasm. (a–c) Western blot analyses of changing levels of RIP140 in cytoplasmic (Cyt) and nuclear (Nuc) fractions of HT22 cells at the indicated time points following treatment with 1 μM thapsigargin (Tg), 2 μM dithiothreitol (DTT) and 5 μM brefeldin A (BFA). The level of RIP140 relative to β-actin (cytoplasmic marker) or laminA/C (nuclear marker) is shown in the lower panel. (d) Confocal microscopy shows representative images of green fluorescence in cultured hippocampal neurons infected with lentivirus carrying GFP–RIP140. Nucleus is labelled with 4′,6-diamidino-2-phenylindole (DAPI) (blue) and arrows point to GFP–RIP140 retained in the nucleus in control, and those exported to the cytoplasm following treatment with 10 μM amyloid-beta (Aβ). Bar graph shows GFP intensity representing RIP140 level. Data from three independent experiments (37 cells from control group and 44 cells from Aβ-treated group) are presented as means±s.e.m.,**P=0.0087,***P=0.00032 compared with control group as determined by Student’st-test. Scale bar, 20 μm. (e,f) Western blot analyses of RIP140 level in Cyt and Nuc of HT22 cells exposed to 1 μM Tg and 2 μM DTT for the durations indicated in the presence of cycloheximide (CHX, 10 μM) to block translation. (g) Western blot analyses of transfected Flag-RIP140 mutant (CN) in different fractions of HT22 cells treated with 1 μM Tg. (h) Western blot analyses of endogenous RIP140 level in Cyt and Nuc of HT22 cells treated with 1 μM Tg following incubation with PKC inhibitor (CHE). Figure 1g confirms that the nuclear export-deficient mutant RIP140 failed to translocate out of the nucleus in Tg-treated cells. Figure 1h further supports this notion because the PKC inhibitor (CHE) blocked nuclear export of RIP140 in Tg-treated cells. These experiments demonstrate that in stressed hippocampal neurons, RIP140 is exported from the nucleus to the cytoplasm via a PKC-mediated nuclear export pathway. Figure 1: UPR induces RIP140 translocation to cytoplasm. ( a – c ) Western blot analyses of changing levels of RIP140 in cytoplasmic (Cyt) and nuclear (Nuc) fractions of HT22 cells at the indicated time points following treatment with 1 μM thapsigargin (Tg), 2 μM dithiothreitol (DTT) and 5 μM brefeldin A (BFA). The level of RIP140 relative to β-actin (cytoplasmic marker) or laminA/C (nuclear marker) is shown in the lower panel. ( d ) Confocal microscopy shows representative images of green fluorescence in cultured hippocampal neurons infected with lentivirus carrying GFP–RIP140. Nucleus is labelled with 4′,6-diamidino-2-phenylindole (DAPI) (blue) and arrows point to GFP–RIP140 retained in the nucleus in control, and those exported to the cytoplasm following treatment with 10 μM amyloid-beta (Aβ). Bar graph shows GFP intensity representing RIP140 level. Data from three independent experiments (37 cells from control group and 44 cells from Aβ-treated group) are presented as means±s.e.m., **P =0.0087, ***P =0.00032 compared with control group as determined by Student’s t -test. Scale bar, 20 μm. ( e , f ) Western blot analyses of RIP140 level in Cyt and Nuc of HT22 cells exposed to 1 μM Tg and 2 μM DTT for the durations indicated in the presence of cycloheximide (CHX, 10 μM) to block translation. ( g ) Western blot analyses of transfected Flag-RIP140 mutant (CN) in different fractions of HT22 cells treated with 1 μM Tg. ( h ) Western blot analyses of endogenous RIP140 level in Cyt and Nuc of HT22 cells treated with 1 μM Tg following incubation with PKC inhibitor (CHE). Full size image Next, to study the distribution of cytoplasmic RIP140, we measured the endogenous RIP140 levels in different subcellular fractions derived from HT22 cells following UPR induced by Tg, dithiothreitol and tunicamycin. These data all show that both endogenous RIP140 (detected by western blot using anti-RIP140 antibody) and exogenous RIP140 (transfected by lentivirus and detected by GFP fluorescence) target ER following ER stress ( Fig. 2 ). 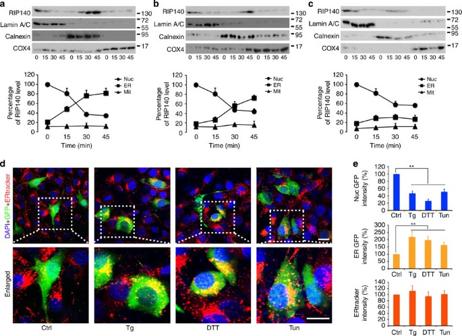Figure 2: UPR induces translocation of RIP140 to the ER. (a–c) Western blot analyses of RIP140 levels in nuclear (Nuc), endoplasmic reticulum (ER) and mitochondrial (Mit) fractions of HT22 cells at different time points following treatment with 1 μM thapsigargin (Tg) (panela), 2 μM dithiothreitol (DTT) (panelb) or 50 μM tunicmycine (Tm) (panelc). The relative protein level was analysed as a percentage of laminA/C for nuclear, calnexin for ER and COX4 for Mit. The RIP140 level in Nuc of control group was calculated as 100%. (d) Representative confocal microscopy images indicating RIP140 cytoplasmic translocation and localization to ER in HT22 cells after treatment with 1 μM Tg, 2 μM DTT and 50 μM Tm. Green fluorescence indicates infected cells with lentivirus carrying GFP–RIP140. Red fluorescence shows ER tracker. Nuclei are labelled with 4′,6-diamidino-2-phenylindole (DAPI) (blue). Scale bars, 20 μm. (e) Percentage of nuclear and cytoplasmic GFP fluorescence or red fluorescence intensity from three independent experiments (43 cells were included in each group), showing RIP140 and ER intensity, respectively, in treated cells compared with control cells. Results are presented as means±s.e.m.,**P<0.01 compare with control group as determined by Student’st-test. Figure 2: UPR induces translocation of RIP140 to the ER. ( a – c ) Western blot analyses of RIP140 levels in nuclear (Nuc), endoplasmic reticulum (ER) and mitochondrial (Mit) fractions of HT22 cells at different time points following treatment with 1 μM thapsigargin (Tg) (panel a ), 2 μM dithiothreitol (DTT) (panel b ) or 50 μM tunicmycine (Tm) (panel c ). The relative protein level was analysed as a percentage of laminA/C for nuclear, calnexin for ER and COX4 for Mit. The RIP140 level in Nuc of control group was calculated as 100%. ( d ) Representative confocal microscopy images indicating RIP140 cytoplasmic translocation and localization to ER in HT22 cells after treatment with 1 μM Tg, 2 μM DTT and 50 μM Tm. Green fluorescence indicates infected cells with lentivirus carrying GFP–RIP140. Red fluorescence shows ER tracker. Nuclei are labelled with 4′,6-diamidino-2-phenylindole (DAPI) (blue). Scale bars, 20 μm. ( e ) Percentage of nuclear and cytoplasmic GFP fluorescence or red fluorescence intensity from three independent experiments (43 cells were included in each group), showing RIP140 and ER intensity, respectively, in treated cells compared with control cells. Results are presented as means±s.e.m., **P <0.01 compare with control group as determined by Student’s t -test. Full size image Cytoplasmic RIP140 interacts with the IP 3 R Since the elevated cytosolic RIP140 increasingly accumulated on ER following UPR, we then determined the cytoplasmic protein that might bind RIP140 by performing a yeast two-hybrid screen. Using RIP140 as the bait, we identified IP 3 R as a RIP140-interacting protein. We then examined the nature of RIP140 interaction with IP 3 R by monitoring its localization to the ER. 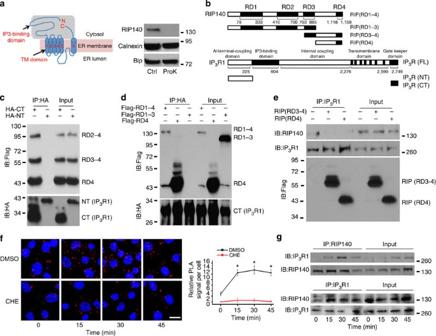Figure 3: RIP140 interacts with IP3R1. (a) Western blot analysis of RIP140 in ER fraction treated with proteinase K (ProK) or without the enzyme (Ctrl). (b) Constructs of RIP140 and IP3R1. (c) Reciprocal coimmunoprecipitation examining the interaction domain of IP3R1 with RIP140. HT22 cells were transfected with HA-tagged N-terminal (NT) or C-terminal (CT) domain of IP3R1 and flag-tagged RD2-4, RD3-4 and RD4 of RIP140. By coimmunopreciping with HA antibody, the flag-tagged domains of RIP140 can be detected only in the presence of CT. (d) Reciprocal coimmunoprecipitation examining the interaction domain of RIP140 with IP3R1. HT22 cells were transfected with HA-tagged C terminus (CT) of IP3R1 and flag-tagged RD1-4, RD4 and RD1-3 of RIP140. By coimmunopreciping with HA antibody, only the RD4-containing flag-tagged RIP140 can be detected. (e) Competition of RD4, or RD4-containing RD(3-4), with the endogenous RIP140 for interacting with IP3R1 in HT22. Cells were transfected with control vector, RD3-4 and RD4, the endogenous IP3R1-interacting RIP140 was detected by RIP140 antibody that can only recognize N-terminal domain of RIP140. RD4 domain of RIP140 competes the binding of RIP140 to IP3R1. (f) Increased association of endogenous RIP140 with IP3R1 monitored byin situPLA assay in HT22 cells treated with thapsigargin for different durations. The red puncta show endogenous RIP140-IP3R1 complexes. The graph shows statistical results presented as means±s.e.m. from five independent experiments;*P<0.05 relative to the control group as determined by Student’st-test. Scale bar, 20 μm. (g) Coimmunoprecipitation examining binding of RIP140 to IP3R1 in HT22 following thapsigargin treatment. Figure 3a shows that RIP140 was detected in the ER fraction but was no longer detectable in the proteinase K-treated ER fraction, in contrast to the intra-membrane protein, calnexin, and the ER lumen protein, Bip, which remained intact following proteinase K treatment. Thus, RIP140 localizes to the outer membrane of the ER. We then determined the interacting domains of RIP140 and IP 3 R in HT22 cells. Figure 3b shows the constructs of RIP140 and IP 3 R used in these reciprocal protein interaction assays. The results of coimmunoprecipitation (co-IP) assays show that RIP140 could be detected only when lysate was co-precipitated with the C-terminal gate-keeping domain of IP 3 R (CT), indicating that CT is the target of RIP140 binding ( Fig. 3c ). A series of truncated mutants of RIP140 were examined for their interaction with IP 3 R-CT in HT22 cells. As show in Fig. 3d , RIP140 mutant lacking RD4 (RD1-3) failed to interact with IP 3 R-CT, suggesting that RD4 of RIP140 is essential and sufficient for its binding to IP 3 R-CT. This finding was further confirmed by in vitro direct protein interaction assays ( Supplementary Fig. 1 ). We then hypothesized that the interaction between RIP140 and IP 3 R might be disrupted by the specific RD4 motif of RIP140. To test this hypothesis, we employed a competitive co-IP assay by overexpressing RD4 in HT22 cells and monitoring the formation of endogenous RIP140/IP 3 R complex using an antibody specific for the N terminus of RIP140 and the IP 3 R antibody ( Fig. 3e ). In the presence of exogenously provided RD4 or RIP140 that contains RD4 (RD3-4), the formation of endogenous RIP140/IP 3 R complex, as indicated by the reciprocally precipitated RIP140 or IP 3 R, was inhibited. Since RD4 of RIP140 is essential and sufficient to mediate the interaction of RIP140 with IP 3 R, we next evaluated the potential function of RD4 motif in response to ER stress. Transfected flag-tagged full-length RIP140 (RD1-4) and RD4 were detected by immunofluorescence assay using flag antibody. As shown in Supplementary Fig. 2 , RD4 was initially homogenously distributed in nuclei and cytoplasm, and remained evenly distributed following ER stress. As predicted, full-length RIP140 was translocated to cytoplasm and interacted with IP 3 R on ER stress. These results show that RD4 can interact with IP 3 R, but it lacks the signal for translocation in response to ER stress. Finally, we used an in situ proximity ligation assay (PLA) to examine the kinetics of endogenous IP 3 R1-RIP140 complex formation during Tg-induced ER stress. This assay employed two antibodies, anti-RIP140 and anti-IP 3 R, followed by the addition of specific oligonucleotides that could be amplified into fluorescent signals [35] . Only when the two antibodies existed in close proximity (<40 nm) could amplification be successful as indicated by fluorescent signals [36] . Thus, the appearance of fluorescent signal indicates the formation and location of the molecular complex containing specific components recognized by IP 3 R and RIP140 antibodies. As shown in Fig. 3f , Tg rapidly induced the formation of endogenous RIP140/IP 3 R1 complex, which was attenuated by pretreating cells with the PKC inhibitor, CHE. The co-IP in Fig. 3g shows the time-dependent formation of the RIP140/IP 3 R1 complex following Tg treatment, in agreement with the time-dependent association described in the PLA assay. These results show that stress promotes RIP140 export from the nucleus to the cytoplasm where it localizes to the ER and binds the gate-keeping domain of IP 3 R via RIP140’s RD4 domain. Figure 3: RIP140 interacts with IP 3 R1. ( a ) Western blot analysis of RIP140 in ER fraction treated with proteinase K (ProK) or without the enzyme (Ctrl). ( b ) Constructs of RIP140 and IP 3 R1. ( c ) Reciprocal coimmunoprecipitation examining the interaction domain of IP 3 R1 with RIP140. HT22 cells were transfected with HA-tagged N-terminal (NT) or C-terminal (CT) domain of IP 3 R1 and flag-tagged RD2-4, RD3-4 and RD4 of RIP140. By coimmunopreciping with HA antibody, the flag-tagged domains of RIP140 can be detected only in the presence of CT. ( d ) Reciprocal coimmunoprecipitation examining the interaction domain of RIP140 with IP 3 R1. HT22 cells were transfected with HA-tagged C terminus (CT) of IP 3 R1 and flag-tagged RD1-4, RD4 and RD1-3 of RIP140. By coimmunopreciping with HA antibody, only the RD4-containing flag-tagged RIP140 can be detected. ( e ) Competition of RD4, or RD4-containing RD(3-4), with the endogenous RIP140 for interacting with IP 3 R1 in HT22. Cells were transfected with control vector, RD3-4 and RD4, the endogenous IP 3 R1-interacting RIP140 was detected by RIP140 antibody that can only recognize N-terminal domain of RIP140. RD4 domain of RIP140 competes the binding of RIP140 to IP 3 R1. ( f ) Increased association of endogenous RIP140 with IP 3 R1 monitored by in situ PLA assay in HT22 cells treated with thapsigargin for different durations. The red puncta show endogenous RIP140-IP 3 R1 complexes. The graph shows statistical results presented as means±s.e.m. from five independent experiments; *P <0.05 relative to the control group as determined by Student’s t -test. Scale bar, 20 μm. ( g ) Coimmunoprecipitation examining binding of RIP140 to IP 3 R1 in HT22 following thapsigargin treatment. Full size image RIP140 attenuates ER Ca 2+ release in neurons Because RIP140 translocated to the ER in response to stress and interacted with the IP 3 R, we suspected that RIP140 might regulate IP 3 R function. To examine this possibility, primary hippocampal neurons were transfected with plasmids encoding DsRed2 plus RIP140 ( n =7 coverslips, 8 cells) or DsRed2 only ( n =4 coverslips, 4 cells) as an expression control. Non-expressing neurons ( n =11 coverslips, 686 cells) in the same imaging field served as a control ( Fig. 4a–e ). Twenty-four hours after transfection, neurons were loaded with fura-2 and then [Ca 2+ ] i was recorded using digital imaging. Basal [Ca 2+ ] i remained stable in non-expressing neurons and in neurons expressing RIP140 or DsRed2 at 79±3 nM, 68±12 nM and 40±4 nM, respectively. After recording stable basal [Ca 2+ ] i for 1 min, Ca 2+ influx via voltage-gated Ca 2+ channels was evoked by applying a 15-s depolarizing stimulus (50 mM K + ). The depolarization-induced increase in [Ca 2+ ] i was 722±123 nM, 858±366 nM and 606±182 nM for non-expressing neurons, neurons expressing RIP140 and DsRed2, respectively. This transient increase in the [Ca 2+ ] i showed that RIP140 expression did not affect voltage-gated Ca 2+ channel function or [Ca 2+ ] i clearance mechanisms and also served to uniformly load ER Ca 2+ stores [37] . After returning to basal [Ca 2+ ] i , the group I metabotropic glutamate receptor agonist DHPG (30 μM) was superfused for 30 s. Activation of group I metabotropic glutamate receptors activates phospholipase C to generate IP 3 and mobilize ER Ca 2+ in hippocampal neurons [38] . As shown in Fig. 4 , DHPG evoked a rapid increase in [Ca 2+ ] i that quickly returned to basal [Ca 2+ ] i in the maintained presence of the agonist. A secondary response was observed in some cells, which is consistent with IP 3 -evoked [Ca 2+ ] i oscillations described for these cells [39] . Expression of RIP140 attenuated DHPG-evoked Ca 2+ release relative to non-expressing neurons or neurons expressing DsRed2. To confirm that DHPG was evoking Ca 2+ release via activation of the IP 3 R, we applied DHPG in the presence of the IP 3 R antagonist, xestospongin C (10 μM). DHPG-evoked Ca 2+ release was blocked by xestospongin C ( n =5 coverslips, 168 cells) relative to untreated control ( n =3 coverslips, 155 cells; data not shown). We next examined the role of RIP140 in regulating the release of Ca 2+ from ER stores in the HT22 cell line that was used for the preceding translocation and biochemical studies. Tg-evoked Ca 2+ release was recorded from HT22 cells expressing RIP140 ( n =3 coverslips, 114 cells) or a RIP140 mutant (RIP140 RD4-neg) ( n =4 coverslips, 169 cells) that lacks the IP 3 R-binding domain ( Fig. 4f,g ). Non-expressing cells ( n =12 coverslips, 779 cells) served as a control. Basal [Ca 2+ ] i remained stable in non-expressing cells and cells expressing RIP140 or RIP140 (RD4-neg) at 85±2 nM, 101±2 nM and 109±5 nM, respectively. After recording stable basal [Ca 2+ ] i for 5 min, ER Ca 2+ release was evoked by applying Tg (1 μM). Tg evoked a transient increase in [Ca 2+ ] i that returned to basal levels in the maintained presence of the drug. Expression of RIP140 attenuated Tg-evoked Ca 2+ release relative to non-expressing cells or cells expressing RIP140 (RD4-neg). Taken together, these data indicate that RIP140 attenuates ER Ca 2+ release in hippocampal neurons and in HT22 cells via an IP 3 R-dependent mechanism and in a manner dependent on its RD4 domain, respectively. 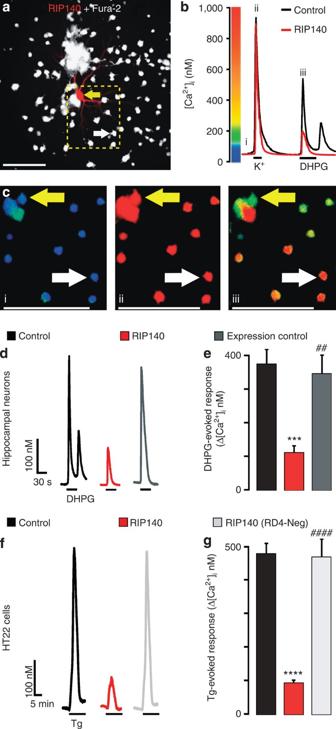Figure 4: RIP140 attenuates ER Ca2+release in neurons. [Ca2+]iwas recorded using fura-2-based digital imaging (Methods). (a) Representative image (n=1 of 8) shows a neuron expressing RIP140 (yellow arrows) and DsRed2 in a field of neurons loaded with fura-2 (white arrows) (scale bar, 100 μm). Neuronal processes are not visible in the fura-2 image because it was focused to the centre of the soma above the focal plane of the dendrites. (b) Representative trace shows [Ca2+]ifor the non-expressing (black) and RIP140-expressing (red) neurons identified by the arrows ina. Neurons were superfused with 50 mM K+and 30 μM DHPG at the times indicated by the horizontal bars inb. (c) Pseudocolour images were scaled as shown inb. Images were collected at the times indicated by the lowercase numerals annotating the traces inb. (d) Representative traces show DHPG-evoked Ca2+release from non-expressing neurons (black) and neurons expressing DsRed2 (dark grey) or RIP140 (red). (e) Bar graph shows net [Ca2+]iincrease evoked by DHPG in non-expressing neurons (black) and neurons expressing DsRed2 (dark grey) or RIP140 (red). ***P<0.001 relative to non-expressing control;##P<0.01 relative to RIP140 as determined by one-way analysis of variance with three levels followed by Tukey’s post test for multiple comparisons. (f) Representative traces show Ca2+release evoked by 1 μM thapsigargin from non-expressing (black) HT22 cells and from HT22 cells expressing RIP140 (red) or RIP140 (RD4-neg) (light grey). (g) Bar graph shows net [Ca2+]iincrease evoked by Tg in non-expressing (black) HT22 cells and HT22 cells expressing RIP140 (red) or RIP140 (RD4-neg) (light grey). ****P<0.0001 relative to control;####P<0.0001 relative to RIP140 as determined by one-way analysis of variance with three levels followed by Tukey’s post test for multiple comparisons. Figure 4: RIP140 attenuates ER Ca 2+ release in neurons. [Ca 2+ ] i was recorded using fura-2-based digital imaging (Methods). ( a ) Representative image ( n =1 of 8) shows a neuron expressing RIP140 (yellow arrows) and DsRed2 in a field of neurons loaded with fura-2 (white arrows) (scale bar, 100 μm). Neuronal processes are not visible in the fura-2 image because it was focused to the centre of the soma above the focal plane of the dendrites. ( b ) Representative trace shows [Ca 2+ ] i for the non-expressing (black) and RIP140-expressing (red) neurons identified by the arrows in a . Neurons were superfused with 50 mM K + and 30 μM DHPG at the times indicated by the horizontal bars in b . ( c ) Pseudocolour images were scaled as shown in b . Images were collected at the times indicated by the lowercase numerals annotating the traces in b . ( d ) Representative traces show DHPG-evoked Ca 2+ release from non-expressing neurons (black) and neurons expressing DsRed2 (dark grey) or RIP140 (red). ( e ) Bar graph shows net [Ca 2+ ] i increase evoked by DHPG in non-expressing neurons (black) and neurons expressing DsRed2 (dark grey) or RIP140 (red). *** P <0.001 relative to non-expressing control; ## P <0.01 relative to RIP140 as determined by one-way analysis of variance with three levels followed by Tukey’s post test for multiple comparisons. ( f ) Representative traces show Ca 2+ release evoked by 1 μM thapsigargin from non-expressing (black) HT22 cells and from HT22 cells expressing RIP140 (red) or RIP140 (RD4-neg) (light grey). ( g ) Bar graph shows net [Ca 2+ ] i increase evoked by Tg in non-expressing (black) HT22 cells and HT22 cells expressing RIP140 (red) or RIP140 (RD4-neg) (light grey). **** P <0.0001 relative to control; #### P <0.0001 relative to RIP140 as determined by one-way analysis of variance with three levels followed by Tukey’s post test for multiple comparisons. Full size image RIP140 suppresses the ‘head-tail’ interaction of IP 3 R It is well established that binding of IP 3 to the IP 3 R promotes a ‘head–tail’ interaction in which the cytoplasmic amino- and carboxyl-termini interact, resulting in channel opening [40] . Since RIP140 bound to the C-terminal gate-keeper domain of IP 3 R and inhibited IP 3 -induced Ca 2+ release without altering IP 3 binding to IP 3 R ( Supplementary Fig. 3 ), we hypothesized that RIP140 might inhibit the ‘head–tail’ interaction of the IP 3 R. We first tested this notion using recombinant proteins in in vitro competition assays, and asked if RD4 domain could prevent IP 3 R-NT from binding to IP 3 R-CT. As shown in Fig. 5a , immunoprecipitation of HA-tagged IP 3 R-CT pulled down flag-tagged IP 3 R-NT. Adding RD4 domain (in various concentrations, +and ++) increasingly abolished IP 3 R-CT interaction with IP 3 R-NT. On the contrary, adding the same amount of RIP140 RD1-3 domain failed to inhibit IP 3 R-CT binding to IP 3 R-NT. Thus, RD4 of RIP140 can inhibit IP 3 R-CT binding to IP 3 R-NT in a dose-dependent manner. Since RIP140 cytoplasmic translocation is the early response to ER stress, cytoplasmic localized RIP140 may act to disrupt IP 3 R-CT and NT interaction. This was confirmed by co-IP assay in HT22 cells that, overexpressing mutant RIP140 (CN), which cannot translocate to cytoplasm, failed to inhibit IP 3 R-CT and -NT interaction ( Fig. 5b ). To examine the ‘head–tail’ interaction of endogenous IP 3 R, we overexpressed or silenced endogenous RIP140, and employed in situ PLA assay to follow the endogenous IP 3 R’s ‘head–tail’ interaction using antibodies against the N-terminal and the C-terminal gate region of IP 3 R. As shown in Fig. 5c,d , in both control transfections (SiCtrl and Vector), m-3M3FBS (m-3M3), which increases IP 3 levels by activating phospholipase C, increased the number of fluorescent puncta indicative of positive ‘head–tail’ interaction resulting from the activation of endogenous IP 3 R. The increased fluorescent puncta were further enhanced following RIP140 knockdown ( Fig. 5c ), but were blocked on RIP140 overexpression ( Fig. 5d ). 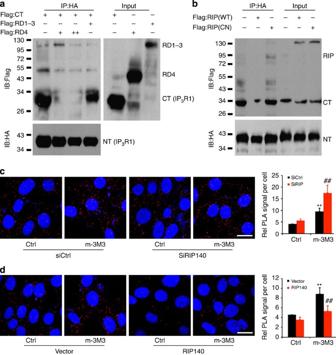Figure 5: RIP140 interrupts ‘head–tail’ interaction of IP3R. (a)In vitrocompetition assay using RD4 to compete out the binding of IP3R1-NT to IP3R1-CT. RIP140 RD1-3 was used as a negative control. Inputs correspond to 10% of flag-labelled protein as indicated. The binding of IP3R-NT to IP3R-CT was significantly blocked by an increasing concentration (++) of RD4. (b) Coimmunoprecipitation examining the effect of cytoplasmic RIP140 on IP3R1 ‘head–tail’ interaction. HT22 cells were transfected with HA-tagged C terminus (CT) and flag-tagged N terminus (NT) of IP3R1 and flag-tagged wild-type RIP140 (WT) or mutant RIP140 (CN), which is localized in the nucleus. Only expressing WT RIP140, but not the mutant (CN), blocked IP3R1-CT and NT interaction. (c,d) The ‘head–tail’ interaction of endogenous IP3R1 was examined in HT22 cells.In situPLA assay was used to monitor the interaction of endogenous IP3R1’s ‘head’ (N-terminal-suppressing domain) and ‘tail’ (C-terminal gate-keeper domain) using antibodies specific to C or N terminus of IP3R1. Red puncta show positive ‘head–tail’ interaction of endogenous IP3R1. ‘Head–tail’ interaction was increased by applying the PLC activator m-3M3FBS (10 μM; m-3M3). The increased ‘head–tail’ interaction was further enhanced following RIP140 knockdown (c) and was abolished on RIP140 overexpression (d). The statistic results of ‘head–tail’ interaction from three independent experiments (seven different fields from each experiment) are presented as means±s.e.m.,**P<0.01 compare with control group;##P<0.01 reletive to SiCtrl or Vector as determined by one-way analysis of variance. Scale bar, 20 μm. These data show that RIP140 negatively regulates IP 3 R-mediated channel opening by interfering with the ‘head–tail’ interaction of IP 3 R. Figure 5: RIP140 interrupts ‘head–tail’ interaction of IP 3 R. ( a ) In vitro competition assay using RD4 to compete out the binding of IP 3 R1-NT to IP 3 R1-CT. RIP140 RD1-3 was used as a negative control. Inputs correspond to 10% of flag-labelled protein as indicated. The binding of IP 3 R-NT to IP 3 R-CT was significantly blocked by an increasing concentration (++) of RD4. ( b ) Coimmunoprecipitation examining the effect of cytoplasmic RIP140 on IP 3 R1 ‘head–tail’ interaction. HT22 cells were transfected with HA-tagged C terminus (CT) and flag-tagged N terminus (NT) of IP 3 R1 and flag-tagged wild-type RIP140 (WT) or mutant RIP140 (CN), which is localized in the nucleus. Only expressing WT RIP140, but not the mutant (CN), blocked IP 3 R1-CT and NT interaction. ( c , d ) The ‘head–tail’ interaction of endogenous IP 3 R1 was examined in HT22 cells. In situ PLA assay was used to monitor the interaction of endogenous IP 3 R1’s ‘head’ (N-terminal-suppressing domain) and ‘tail’ (C-terminal gate-keeper domain) using antibodies specific to C or N terminus of IP 3 R1. Red puncta show positive ‘head–tail’ interaction of endogenous IP 3 R1. ‘Head–tail’ interaction was increased by applying the PLC activator m-3M3FBS (10 μM; m-3M3). The increased ‘head–tail’ interaction was further enhanced following RIP140 knockdown ( c ) and was abolished on RIP140 overexpression ( d ). The statistic results of ‘head–tail’ interaction from three independent experiments (seven different fields from each experiment) are presented as means±s.e.m., **P <0.01 compare with control group; ## P <0.01 reletive to SiCtrl or Vector as determined by one-way analysis of variance. Scale bar, 20 μm. Full size image RIP140-IP 3 R interaction protects neurons against ER stress Considering that stress promotes translocation of RIP140 to the cytoplasm to interact with the IP 3 R and that overexpressing RIP140 attenuates IP 3 R-mediated Ca 2+ release, we speculated that the cytoplasmic RIP140 might protect cells from ER stress. To examine this notion, we inhibited the interaction of RIP140 with IP 3 R and then measured the ER stress response in HT22 cells. Several strategies were used to inhibit RIP140 interaction with IP 3 R including: siRNA-mediated knockdown of RIP140 (SiRIP140), expressing a mutant RIP140 that is deficient in nuclear export (CN) or expressing a truncation mutant of RIP140 that lacks the RD4 domain (RD1-3). 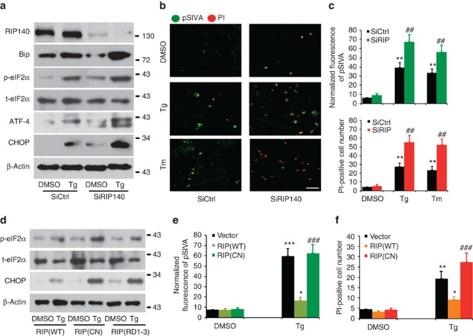Figure 6: Interaction of RIP140 with IP3R is required for its protective role against ER stress. (a) Western blot analyses of ER stress-related protein levels in control (SiCtrl) or RIP140 knockdown (SiRIP140) HT22 cells treated with 1 μM thapsigargin (Tg) for 3 h. (b) Apoptotic cells were detected by pSIVA–PI-positive staining in HT22 transfected with siRNA against RIP140 (SiRIP140) and treated with Tg or Tm for 3 h. Representative image of green fluorescence shows pSIVA staining and red fluorescence shows propidium iodide (PI). Scale bar, 40 μm. (c) Quantified results of pSIVA intensity and PI-positive cell number. (d) Western blot analyses of ER stress-related proteins in response to Tg treatment in HT22 cells transfected with wild type (WT) or mutated RIP140 (CN) and RIP1-3 of RIP140 (RIP1-3). (e,f) Quantified results of apoptotic cells detected by pSIVA (e) and PI-positive (f) staining in HT22 cells expressing wild type (WT) or mutated RIP140 (CN) following treatment with Tg for 3 h. The pSIVA intensity and PI-positive cell number from seven different fields per group of three independent experiments are presented as means±s.e.m.,*P<0.05,**P<0.01 and***P<0.001 relative to dimethylsulphoxide (DMSO) control group;##P<0.01,###P<0.001 reletive to treated SiCtrl and WT RIP140 transfected group as determined by one-way analysis of variance, respectively. Figure 6a shows that Tg induced ER stress in the control cell (SiCtrl) as indicated by upregulated expression of Bip, ATF4, CHOP and phosphorylated eIF2a. These stress-induced changes were enhanced by knockdown of RIP140 (SiRIP140). In consistence with this observation, treatment of cultured hippocampal neurons with aggregated Aβ peptide increased the expression of CHOP, and the level of CHOP was further elevated in RIP140-deficit neurons ( Supplementary Fig. 4 ). These results indicate that RIP140 plays a protecting role against Aβ neurotoxicity. To validate the neuroprotective effect of RIP140 against stress-induced apoptosis, we monitored cell apoptosis by pSIVA–propridium iodide (PI) double staining. pSIVA detects cell surface phosphatidylserine, an early marker for apoptosis, and PI labels the nuclei of dead cells. Figure 6b,c show that knockdown of RIP40 increased ER stress resulting in an increased number of cells labelled for pSIVA and PI. Importantly, Fig. 6d shows that expressing the mutant RIP140 (CN- and RD4-deleted RIP140) increased the extent of ER stress relative to expressing wild-type RIP140 (RIP140-WT), as indicated by the elevation of ER stress markers phosphorylated eIF2α (p-eIF2α) and CHOP. Furthermore, compared with wild-type RIP140, mutant RIP140 (RIP140-CN) failed to protect cells from ER stress-induced apoptosis ( Fig. 6e,f ). These results demonstrate that RIP140 protects cells from ER stress. Figure 6: Interaction of RIP140 with IP 3 R is required for its protective role against ER stress. ( a ) Western blot analyses of ER stress-related protein levels in control (SiCtrl) or RIP140 knockdown (SiRIP140) HT22 cells treated with 1 μM thapsigargin (Tg) for 3 h. ( b ) Apoptotic cells were detected by pSIVA–PI-positive staining in HT22 transfected with siRNA against RIP140 (SiRIP140) and treated with Tg or Tm for 3 h. Representative image of green fluorescence shows pSIVA staining and red fluorescence shows propidium iodide (PI). Scale bar, 40 μm. ( c ) Quantified results of pSIVA intensity and PI-positive cell number. ( d ) Western blot analyses of ER stress-related proteins in response to Tg treatment in HT22 cells transfected with wild type (WT) or mutated RIP140 (CN) and RIP1-3 of RIP140 (RIP1-3). ( e , f ) Quantified results of apoptotic cells detected by pSIVA ( e ) and PI-positive ( f ) staining in HT22 cells expressing wild type (WT) or mutated RIP140 (CN) following treatment with Tg for 3 h. The pSIVA intensity and PI-positive cell number from seven different fields per group of three independent experiments are presented as means±s.e.m., *P <0.05, **P <0.01 and ***P <0.001 relative to dimethylsulphoxide (DMSO) control group; ## P <0.01, ### P <0.001 reletive to treated SiCtrl and WT RIP140 transfected group as determined by one-way analysis of variance, respectively. Full size image Loss of RIP140 enhances ER stress-induced neuronal death To validate the functional role for RIP140 in protecting neurons from ER stress in vivo , we employed an animal model of ER stress induced by intraperitoneal injection of Tg [41] . Lentivirus carrying shRNA against RIP140 was injected stereotaxically to knock down endogenous RIP140 in the CA1 region of the hippocampus as depicted in Fig. 7a . 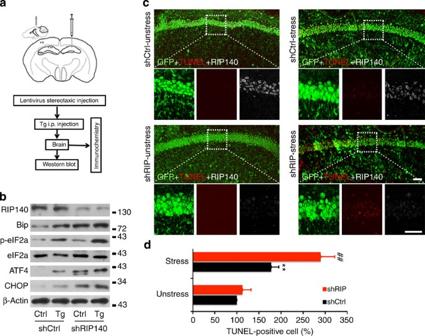Figure 7: RIP140 protects cells from ER stress in mouse brain. (a) Cartoon depicting the site of lentiviral injection and the experimental procedure. (b) Western blot analyses of RIP140 and ER stress-related proteins Bip, p-eIF2a, ATF4 and CHOP in the virus-injected brain area 5 days after injection with lentivirus-ShRIP140 (lenti-ShRIP140) or lentivirus-control (lenti-Ctrl). (c) TUNEL staining (red puncta) of brain sections from the lentivirus-infected areas 20 days after virus injection (2 days post stress induction). 4',6-diamidino-2-phenylindole (DAPI) (blue) depicts nuclear staining and green signals show lentivirus-infected cells. Scale bar, 20 μm. (d) Bar graph shows the percentage of TUNEL-positive cells versus total cell number from same field. The results from five different fields in each group are presented as means±s.e.m.,**P<0.01 compare with unstressed group;##P<0.01 relative to stressed lenti-Ctrl group as determined by one-way analysis of variance. Figure 7b (top) and Supplementary Fig. 5 confirmed the reduction in RIP140 protein level in animals injected with shRNA against RIP140 (shRIP140). ER stress was elicited 3 or 18 days after lentivirus delivery of shRNA, and analyses of the hippocampus were conducted 2 days later. Figure 7b (panels 2–6) show elevated ER stress-related proteins, including Bip, phosphorylated eIF2a (p-eIF2a), ATF4 and CHOP in Tg-treated control (without silencing RIP140) animals. The RIP140-silenced animals (shRIP140, 5 days post lentivirus injection), even without Tg induction, exhibited elevated ER stress markers that were enhanced by treatment with Tg. Cells from RIP140 knockdown mice (20 days post lentivirus injection) exhibited increased apoptosis on Tg treatment ( Fig. 7c,d ). These animal studies validate a functional role for RIP140 in neuroprotection against ER stress in vivo . Figure 7: RIP140 protects cells from ER stress in mouse brain. ( a ) Cartoon depicting the site of lentiviral injection and the experimental procedure. ( b ) Western blot analyses of RIP140 and ER stress-related proteins Bip, p-eIF2a, ATF4 and CHOP in the virus-injected brain area 5 days after injection with lentivirus-ShRIP140 (lenti-ShRIP140) or lentivirus-control (lenti-Ctrl). ( c ) TUNEL staining (red puncta) of brain sections from the lentivirus-infected areas 20 days after virus injection (2 days post stress induction). 4',6-diamidino-2-phenylindole (DAPI) (blue) depicts nuclear staining and green signals show lentivirus-infected cells. Scale bar, 20 μm. ( d ) Bar graph shows the percentage of TUNEL-positive cells versus total cell number from same field. The results from five different fields in each group are presented as means±s.e.m., **P <0.01 compare with unstressed group; ## P <0.01 relative to stressed lenti-Ctrl group as determined by one-way analysis of variance. Full size image RIP140 is highly expressed in metabolic tissues and the brain. The physiological role for RIP140 in metabolism is primarily mediated by its nuclear receptor co-regulator activity that regulates insulin sensitivity and inflammatory responses in adipocytes and macrophages [31] . How RIP140 may function in the brain has not been determined. This study reveals rapid nuclear export of RIP140 to the cytoplasm in ER-stressed hippocampal neurons. The study also reports a new functional role for cytoplasmic RIP140 in neurons. RIP140 attenuates ER stress by interacting with IP 3 R through the carboxyl-terminal RD4 domain of RIP140 and the C-terminal gate-keeping domain of the IP 3 R. This interaction interferes with IP 3 R’s ‘head–tail’ interaction, thereby suppressing Ca 2+ release and preventing neuronal death. Finally, the physiological relevance of this novel protective mechanism against Aβ neurotoxicity and ER stress was demonstrated in hippocampal neuron cultures and an animal model. Our previous studies showed a specific signalling pathway regulating the phosphorylation of RIP140, which triggers nuclear export of RIP140 in adipocytes [26] . The signalling pathway is initiated by activated nuclear PKCε, which specifically phosphorylates Ser 102 and Ser 1003 of RIP140, followed by arginine methylation on Arg 240 , Arg 650 and Arg 948 (ref. 34 ). PKCε is broadly expressed in neuronal tissue and is regarded as a stress sensor [42] , [43] . Increased cytosolic Ca 2+ causes PKCε activation, which plays protective roles against hypoxia and excitatory neurotoxicity [44] . Interestingly, activation of PKCε protects neurons from ER stress-induced apoptosis [45] . In the present study, hippocampal neurons appear to engage the PKCε-dependent pathway to stimulate RIP140’s nuclear export on ER stress. Both inhibiting PKCε and mutating RIP140 to abrogate its PKC-elicited nuclear export can abolish the protective function of RIP140 in stressed neurons. Of significance is the observation that acute ER stress readily triggers nuclear export of RIP140 in hippocampal neurons, which can be a new signalling pathway mediating PKCε action as a stress sensor to protect neurons from ER stress-induced cell death. This may represent a fundamental, stress-elicited physiological mechanism to rapidly resolve acute ER stress in neurons. However, it remains to be determined whether this may provide any protection during chronic ER stress. The fate of the exported RIP140 following its binding to the IP 3 R also awaits further study. With respect to the molecular mechanism, it is known that IP 3 R activity is controlled by the direct association of its head and tail in both homo- and hetero-tetrameric complexes [12] , [40] , [46] . Interestingly, this can be regulated by RIP140 via a direct interaction with the IP 3 R C-terminal gate-keeper domain, which disrupts the ‘head–tail’ interaction and then suppresses channel opening and Ca 2+ release. Importantly, a simple RD4 epitope is sufficient to reduce the formation of endogenous RIP140/IP 3 R complex. Thus, the RIP140 RD4 domain interaction with the C-terminal gate-keeper domain of the IP 3 R may serve as a potential therapeutic target in diseases related to ER stress. ER homoeostasis is regulated by Ca 2+ uptake and efflux through various transporters and ion channels on the ER membrane that are modulated by intracellular signalling cascades [47] , [48] . Depleting the ER Ca 2+ store by blocking ER membrane Ca 2+ pumps or through uncontrolled ER Ca 2+ release results in ER stress and cell death, which is believed to contribute to the development of neurodegenerative disease [49] , [50] . Activating IP 3 Rs is known to trigger pathological processes, including apoptosis [51] . A recent study showed that loss of IP 3 R1 enhances neuronal vulnerability to ER stress via a mitochondria-dependent pathway in an animal model [52] . Furthermore, stimulation of ER Ca 2+ release channels accelerates Tg-induced ER depletion and apoptosis [53] and reducing Ca 2+ release from ER by pharmacologically blocking IP 3 R-mediated Ca 2+ release following treatment with a sarcoendoplasmic reticulum calcium transport ATPase inhibitor-attenuated ER stress and improved cell survival [8] . These studies demonstrate complicated regulation of IP 3 R in normal and stressed conditions. Despite an in-depth understanding of IP 3 R activation by its binding partner [54] , much less is known about the negative regulation of the IP 3 R. The present study describes a new physiological pathway, initiated by ER stress, in which nuclear export of RIP140 provides an immediate negative regulatory mechanism to attenuate IP 3 R activity and the subsequent stress response. While RIP140 does not seem to affect IP 3 binding to IP 3 R ( Supplementary Fig. 3 ), it remains to be determined whether and how RIP140 may affect the action of other IP 3 R regulatory molecules implicated in the regulation of IP 3 R-mediated Ca 2+ release, such as cytochrome c and bcl-2 (refs 55 , 56 ). IP 3 R-mediated Ca 2+ release is regulated by IP 3 R modulatory proteins that can act on either cytosolic or luminal sites [17] , [57] . Intralumenal proteins, such as ERp44 and chromogranin, are typically involved in long-term chronic stress [58] . Ca 2+ -dependent apoptosis is regulated by ER oxidase 1-a that disrupts the interaction between ERp44 and IP 3 R in prolonged ER stress [59] . Interaction of the IP 3 R with cytosolic proteins, like cytochrome c and bcl-2, represents a delayed response following ER stress [17] , [60] . RIP140 is a different type of cytosolic regulator of the IP 3 R because it acts by rapidly attenuating the IP 3 R ‘head–tail’ interaction immediately following stress induction. How this newly identified mechanism may be integrated with other IP 3 R modulatory events to maintain the homoeostasis of IP 3 R activity remains to be determined. Cell cultures Primary hippocampal neurons were isolated as previously described [61] . Briefly, the hippocampal tissues from embryonic (E16-18) mice brain were dissociated with 0.25% trypsin and cultured on poly-d-lysine-coated plates in neurobasal medium supplemented with B27. The experiments were carried after 12–14 days of culture (DIV 12–14). HT22 cells (from Salk Institute) were maintained with Dulbecco’s modified eagles medium supplemented with 10% fetal bovine serum and differentiated in neurobasal medium with N2 supplement for 3 days before treatment. [Ca 2+ ] i imaging Intracellular Ca 2+ concentration ([Ca 2+ ] i ) was recorded as previously described [62] with minor modifications. Cells (DIV12-14) were loaded with fura-2 by incubation in hepes-buffered Hanks’ salt solution containing 5 μM fura-2 acetoxymethyl ester in 0.04% pluronic acid for 30 min at 37 °C followed by washing in the absence of indicator for 10 min. Coverslips containing fura-2-loaded cells were transferred to a recording chamber, placed on the stage of an Olympus IX71 microscope (Melville, NY, USA), and viewed through a × 20 objective. Excitation wavelength was selected with a galvanometer-driven monochromator (8-nm slit width) coupled to a 75-W xenon arc lamp (Optoscan; Cairn Research). [Ca 2+ ] i was monitored using sequential excitation of fura-2 at 340 and 380 nm; image pairs were collected every 1 s. For experimental recordings, cells were superfused at a rate of 1–2 ml min −1 with hepes-buffered Hanks’ salt solution for 2 min followed by a 15-s perfusion of 50 mM K + to depolarize the neurons and equally load the ER with Ca 2+ . Ca 2+ release from IP 3 -sensitive stores was evoked by 30-s superfusion with 30 μM (S)-3,5-dihydroxyphenylglycine (DHPG). Ca 2+ release from the ER of HT22 cells was evoked by Tg diluted in hepes-buffered Hanks’ salt solution and bath applied to a final concentration of 1 μM. Fluorescence images (510/40 nm) were projected onto a cooled charge-coupled device camera (Cascade 512B; Roper Scientific) controlled by MetaFluor software (Molecular Devices). After background subtraction, the 340- and 380-nm image pairs were converted to [Ca 2+ ] i using the formula [Ca 2+ ] i = K d β ( R − R min )/( R max − R ) where R is 340/380 nm fluorescence intensity ratio. The dissociation constant used for fura-2 was 145 nM, and β was the ratio of fluorescence intensity acquired with 380-nm excitation measured in the absence and presence of Ca 2+ . R min , R max and β were determined in a series of calibration experiments on intact cells by applying 10 μM ionomycin in Ca 2+ -free buffer (1 mM ethylene glycol tetraacetic acid (EGTA)) and saturating Ca 2+ (5 mM Ca 2+ ). Values for R min , R max and β were 0.37, 9.38 and 6.46, respectively. These calibration constants were applied to all experimental recordings. The neuronal cell body was selected as the region of interest for all recordings. All neurons within imaging fields were included in the analysis and no exclusions were made. To generate pseudocolour images, a binary mask was generated by applying an intensity threshold to the 380-nm image and applied to [Ca 2+ ] i images with colours assigned as indicated by the calibration bars in the figures. Plasmids and siRNAs Flag- or HA-tagged full-length and truncated constructs of RIP140 corresponding to different lengths (see Fig. 3b ) were generated by PCR from mouse cDNA and subcloned into the site of Bam HI and Nhe I of pCMX-PL1 (System Biosciences). The primers for RIP140 are: 5′-GGCAGCAAACCTGAATTCGGC-3′ (sense), 5′-CTCACCGGGCACGGAACATC-3′ (antisense). cDNA encoding the N-terminal coupling domain (IP 3 R1/NT, aa 1–225) and C-terminal gate-keeping domain of IP 3 R1 (IP 3 R1/CT, aa 2,590–2,749) were generated by PCR from mouse cDNA and subcloned into the site of Eco R1 and Kpn 1 of pCMX-PL1. Constitutive nuclear export negative mutation of RIP140 (CN) involving residues Ser102 and Ser1003 was made using QuikChange XL site-directed mutagenesis kit (Stratagene). The mutagenic primers are: S102A: 5′-CGGAAGAGGCTGGCTGATGCCATCGTG-3′ (sense), 5′-CACGATGGCATCAGCCAGCCTCTTCCG-3′ (antisense); S1003A: 5′-CATAGGACATTTGCATACCCGGGAATG-3′ (sense), 5′-CATTCCCGGGTATGCAAATGTCCTATG-3′ (antisense). Scrambled RNA and siRNAs for Nrip1 (5′-CGGCGTTGACATCAAAGAA-3′ and 5′-GCTTCTTTCTTTAATCTAA-3′, SI02698759) were from Qiagen. Lentivirus production, concentration and transduction Full-length RIP140 or shRIP140 (target sequence: 5′-CCCGGCGTTGACATCAAAGAA-3′ and 5′-AAGCTTCTTTCTTTAA-3′) was subcloned into the site of Not I and Xba I of pCDH-GFP (System Biosciences) to generate RIP140 overexpression or RIP140-silence lentiviral vectors. Lentivirus was concentrated and titled as described [63] . Briefly, 293T cells were transfected with expression vectors (full-length RIP140 or shRIP140) and packaging vectors (System Biosciences). Lentivirus-containing medium was collected at 24, 48 and 72 h after transfection. Viral particles were concentrated by ultracentrifugation and purified through a sucrose cushion (20% sucrose in HBSS). Concentrated and purified virus was suspended in HBSS and stored at −80 °C. For transduction, neurons were incubated with lentivirus for 16 h and then the medium was replaced with fresh culture medium. Cell transfection Mouse primary hippocampal neurons were transfected between 12–14 days in vitro using a modification of a calcium phosphate protocol. Briefly, hippocampal cultures were incubated for 30 min in Dulbecco’s modified eagles medium supplemented with 1 mM kynurenic acid, 10 mM MgCl 2 and 5 mM HEPES. A DNA/calcium phosphate precipitate containing 1 μg plasmid DNA per well was prepared, allowed to form for 30 min at 21 °C then added to the culture. Following 90-min incubation, cells were washed once with Dulbecco’s modified eagles medium supplemented with MgCl 2 and HEPES and then returned to conditioned media. HT22 cells were transfected with siRNA to knockdown RIP140 using HiPeFect transfect reagent (301707, QIAGEN) according to the manufacturer’s instruction. The plasmid DNA was transfected into HT22 cells using Lipofectamine 2000 Transfection Reagent(11668019, Invitrogen) according to the manufacturer’s instruction. Western blotting For western blotting, the cell lysates were prepared by sonication in RIPA buffer with protease and phosphatase inhibitor cocktails. Proteins (60–80 μg) were separated by 8–15% SDS–polyacrylamide gel electrophoresis gel electrophoresis and transferred to polyvinylidene difluoride membranes, blocked (in 5% milk) and incubated overnight in primary antibodies (information is provided in Supplementary Table 1 ) followed by respective anti-IgG secondary antibodies. Membranes were developed for visualization and photography using ECL reagent (Thermo). Optical band densities were quantified using Pro-Gel Image software and the result was analysed using SPSS17.0 software. Uncropped images of all blots are shown in Supplementary Figs 5–14 . In situ proximal ligation assay In situ proximal ligation assay was performed using Duolink PLA assay kit (Olink Bioscience) according to the protocol provided by the manufacturer. Briefly, cells were fixed using 4% polyparaformaldehyde and incubated with primary antibodies overnight at 4 °C. To detect the endogenous interaction of RIP140 with IP 3 R1, anti-RIP140 (sc-8997; Santa Cruz; 1:200) and anti-IP 3 R (sc-271197; Santa Cruz; 1:200) were used. The IP 3 R1 C- and N-terminal association was detected using antibodies recognize C-(407140, Calbiochem; 1:300) and N terminus(LS-C121863, Lifespan; 1:300) of IP 3 R1. Images were acquired by Olympus FluoView 1000 IX2 upright confocal microscope. The fluorescent puncta represent protein complex from different fields of individual experiment was counted with ImageJ image processing freeware ( http://rsbweb.nih.gov/ij/ ), and the result was analysed using SPSS17.0 software. Subcellular fractionation Subcellular fractions including ER, mitochondria and nuclear from cell or hippocampus were isolated using ER and mitochondria isolation kit (ER 0100 and MITOISO2, Sigma) according to the protocol. Detection of apoptosis Cell apoptosis was detected using CytoGLO SIVA-IANBD kit (IMG-6701K, IMGENEX) and CF594 terminal dUTP nick end labeling (TUNEL) apoptosis detection kit (30064, Biotium) according to the protocol. Images were acquired by Olympus FluoView 1000 IX2 upright confocal microscope. The fluorescence intensity representing pSIVA, PI and TUNEL-positive cell number from different fields was counted using ImageJ and quantified. Aβ aggregation and cell treatment The aggregation of peptide was described as previously [64] . Briefly, synthetic Aβ 1-40 and Aβ 1-42 (American Peptide, 62-0-86 and 62-0-80) were dissolved to 0.5 mg ml −1 in neurobasal medium and incubated for 4 days at 37 °C. Cultured hippocampal neurons were incubated with 10 μM of aggregated peptide for 24 h and then immunofluorescence was performed. In vitro competition assay HA-tagged IP 3 R-NT was synthesized in vitro using a coupled reticulocyte lysate system(TNT, promega) and incubated overnight at 4 °C with the presence of flag-tagged IP 3 R-CT. Sequential reactions were prepared with increasing amounts of flag-tagged RD4 synthesized in a TNT system present in reaction. Flag-tagged RD1-3 was added to the reaction as negative control. In vitro pull-down assay was then performed and the protein levels of IP 3 R-CT, RD4 and RD1-3 were determined by western blot. Animal experiments Male adult C57BL/6 mice (8–9 weeks old), from Charles River Laboratories, were maintained and experimental procedures were conducted according to NIH guidelines and approved by the University of Minnesota Institutional Animal Care and Use Committee (Protocol no. 1007A86332). Lentivirus carrying RIP140-shRNA was delivered to hippocampus using stereotaxic apparatus at anteroposterior 2.0 mm, medial-lateral 1.2 mm and dorsoventral1.6 mm as previously described [65] . RIP140 protein levels following virus injection were detected using immunofluorescence and western blot as indicated in the figure legend. The ER stress animal models were generated following intraperitoneal injection of Tg (1 μg g −1 ) or normal saline(control) after 3 or 18 days of virus injection. Then the animals were anaesthetised 2 days later and brain tissues were subjected to immunofluorescence staining or protein extraction. To detect the apoptotic cells, TUNEL staining of brain sections was performed using CF594 TUNEL apoptosis detection kit (30064, Biotium). Images were acquired by Olympus FluoView 1000 IX2 upright confocal microscope. The TUNEL-positive cell numnber versus total cell number indicated by 4',6-diamidino-2-phenylindole from the lentivirus-infected areas was counted and quantified. Background was adjusted using ImageJ before counting. Statistical analyses Statistical significance for multiple comparisons was determined by Student’s t -test or analysis of variance as indicated in the figure legend using SPSS17.0 software and summarized as the mean±s.e.m. of repeated measures, P <0.05 was considered statistically significant at the 95% level. For [Ca 2+ ] i imaging studies, an individual experiment ( n =1) was defined as the change in DHPG-evoked or Tg-evoked Ca 2+ release from a single cell on a single coverslip. Changes in DHPG-evoked or Tg-evoked Ca 2+ release are presented as mean±s.e.m. Each experiment was replicated using at least three separate coverslips from at least two separate cultures. Significant differences were determined by one-way analysis of variance with three levels followed by Tukey’s post hoc test for multiple comparisons (OriginPro v8.5). How to cite this article: Feng, X. et al . Receptor-interacting protein 140 attenuates endoplasmic reticulum stress in neurons and protects against cell death. Nat. Commun. 5:4487 doi: 10.1038/ncomms5487 (2014).